Loss-of-function genomic variants highlight potential therapeutic targets for cardiovascular disease Pharmaceutical drugs targeting dyslipidemia and cardiovascular disease (CVD) may increase the risk of fatty liver disease and other metabolic disorders. To identify potential novel CVD drug targets without these adverse effects, we perform genome-wide analyses of participants in the HUNT Study in Norway (n = 69,479) to search for protein-altering variants with beneficial impact on quantitative blood traits related to cardiovascular disease, but without detrimental impact on liver function. We identify 76 (11 previously unreported) presumed causal protein-altering variants associated with one or more CVD- or liver-related blood traits. Nine of the variants are predicted to result in loss-of-function of the protein. This includes ZNF529 :p.K405X, which is associated with decreased low-density-lipoprotein (LDL) cholesterol (P = 1.3 × 10 −8 ) without being associated with liver enzymes or non-fasting blood glucose. Silencing of ZNF529 in human hepatoma cells results in upregulation of LDL receptor and increased LDL uptake in the cells. This suggests that inhibition of ZNF529 or its gene product should be prioritized as a novel candidate drug target for treating dyslipidemia and associated CVD. Cardiovascular disease (CVD) – in particular cerebrovascular and ischemic heart diseases – is the leading cause of death globally [1] . Lowering circulating lipids is an important treatment strategy to reduce risk [2] . However, some pharmaceutical mechanisms of lipid lowering and CVD risk reduction may unfortunately increase risk of fatty liver disease or other metabolic disorders [3] , [4] , [5] , [6] . The vast majority of novel candidate drugs that enter clinical testing fail to demonstrate sufficient safety and efficacy to gain regulatory approval. This is largely due to poor predictive value of preclinical models of disease along with a lack of knowledge about the long-term consequences of targeting specific biological processes in humans [7] . It has been estimated, however, that drugs with genetic support of efficacy are twice as likely to have success in clinical testing [8] . We aim to identify novel candidate pharmaceutical strategies for CVD risk reduction that, importantly, are unlikely to increase the risk of liver disease, diabetes, or other metabolic disorders. To attain this, we conduct a large data-driven genomic discovery effort to identify presumed causal protein-altering variants with impact on lipids and other liver-related blood traits. In particular, we are interested in identifying presumed causal protein-altering variants associated with a more favorable lipid profile without being associated with elevated liver enzymes or vice versa. We analyze 9 liver-related blood traits in close to 70,000 participants in the Trøndelag Health (HUNT) Study. The HUNT Study is a large population-based health survey conducted in a geographically confined region in Norway [9] . The examined traits are related to: (i) blood lipid levels which impact cardiovascular, neurological and eye-related diseases: total cholesterol (TC), low-density lipoprotein cholesterol (LDL-C), high-density lipoprotein cholesterol (HDL-C) and triglyceride (TG) levels; (ii) C-reactive protein (CRP; only values <15 mg/L were included) which is predictive of cardiovascular disease [10] ; and (iii) enzymes which primarily reflect liver function: alanine aminotransferase (ALT), aspartate aminotransferase (AST), alkaline phosphatase (ALP) and gamma-glutamyltransferase (GGT). To maximize chances of discovery of presumed causal protein-altering variants associated with the 9 blood traits, we combine a number of genomic approaches, including (i) low-coverage (5x) whole-genome sequencing (WGS) of a subsample of HUNT Study participants ( N = 2202) to identify region-specific rare variants, (ii) targeted genotyping, also including rare region-specific variants identified by WGS, (iii) deep genotype imputation based on the TOPMed multi-ethnic reference panel consisting of 60,039 deeply sequenced genomes [11] , (iv) genome-wide association analyses (GWAS) in up to 69,479 HUNT Study participants (ranging from 21,528 for AST to 69,479 for TG), followed by (v) stepwise conditional analyses and, for the purpose of further fine-mapping loci identified in HUNT, we perform (vi) trans-ancestry meta-analyses in up to 203,476 people of Norwegian, Japanese, and Sardinian ancestry (ranging from 128,794 for CRP to 203,476 for TC) (see Supplementary Fig. 1 for a study design overview). We assume any protein-altering variant to be likely causally related to the trait of interest if the variant (i) was the most statistically significant variant (lowest P) in a genomic region (i.e., the locus index variant) in any of the GWAS or (ii) if the variant was independently associated with the trait of interest in GWAS stepwise conditional analyses. Genomic discovery of presumed causal protein-altering variants We imputed 26 million genomic variants with sufficient quality and at least 10 minor allele copies into 69,479 participants in the HUNT Study (Supplementary Data 1 ). Using a linear mixed model [12] to account for relatedness among study participants, we tested for genome-wide association ( P < 5 × 10 −8 ) with 9 liver-related blood traits. We identified 201 genomic regions (i.e., loci) associated with one or more of the traits. At 24 of the 201 loci, the locus index variant alters ( n = 22) or results in loss-of-function (LoF) ( n = 2) of the protein. We consider these 24 variants as presumed causally related to the trait of interest (Supplementary Fig. 2 and Supplementary Data 2 ). Stepwise conditional analyses resulted in identification of an additional 150 independently associated variants within the 201 loci. These include 28 additional protein-altering variants, hereof 2 LoF variants, which are significantly and independently associated with one or more of the liver-related blood traits (Supplementary Data 3 ). For the purpose of further fine-mapping of loci and identification of additional presumed causal protein-altering variants, we performed trans-ancestry meta-analyses by combining summary statistics based on the primary discovery effort in HUNT with additional GWAS statistics from Sardinia (SardiNIA cohort) [13] and Japan (Biobank Japan) [14] . The combined meta-analyses comprised up to 203,476 participants ( N range 128,794 for CRP to 203,476 for TC) and 31.5 million unique variants ( n range 24.7–31.5 million) (Supplementary Fig. 3 ). The analyses resulted in identification of an additional 86 loci and 351 independent variants, including 13 presumed causal protein-altering variants. 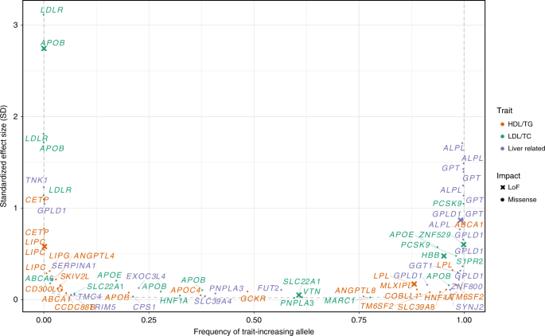Fig. 1: Protein-altering variants with effect on lipid and liver-related blood traits. Smile plot comparing the frequency of the blood-trait increasing allele with the allele’s effect size for protein-altering variants significantly (P< 5 × 10−8) associated with a lipid (HDL-C, LDL-C, TG, TC) or liver (ALT, ALP, AST, GGT) trait. The most significant trait is shown for variants with significant association for multiple traits. Color indicates the trait category for which the variant is significant, with loss-of-function variants shown as x. Power curve (dashed line) denotes estimated 90% power in the meta-analysis with a sample size ofN= 210,000 at alpha = 5 × 10−8. One of the protein-altering variants comprise a previously reported LoF variant in HBB (p.Q40X) [15] associated with decreased TC (Table 1 and Supplementary Data 4 ). Table 1 Loss-of-function variants associated with liver-related blood traits. Full size table To identify rare HUNT-specific presumed causal protein-altering variants, we performed genome-wide association testing for the 9 liver-related blood traits in up to 57,060 HUNT Study participants ( N range 15,520 for AST to 57,060 for TG) based on directly genotyped variants that were included as custom content on the array and not part of the primary GWAS (see Materials and Methods for details). In brief, variants were selected for custom content genotyping if they were (i) identified by HUNT-specific low-coverage (5x) WGS ( N = 2202 HUNT Study participants), (ii) observed in Norwegian clinics for familial hypercholesterolemia, or (iii) not-previously-observed variants predicted to introduce a premature stop codon in any of 56 genes in which protein-altering variants are deemed clinically actionable by The American College of Medical Genetics and Genomics (ACMG56) [16] . This resulted in identification of an additional 11 protein-altering variants, including 4 LoF variants, which are associated with one or more of the 9 traits. Five of the 11 variants originated from region-specific WGS and all variants are rare (ranging from 1 in 178 to 1 in 6313 individuals) (Table 1 and Supplementary Data 5 ). Combining all discovery strategies, we identified a total of 674 unique independent variants within 287 loci associated with at least one of the 9 quantitative liver-related blood traits. Of the 287 loci, 92 have not previously been associated with the trait of interest (Supplementary Fig. 4 ). We identified genome-wide significant associations with at least one trait at 76 presumed causal protein-altering variants, of which 9 result in loss-of-function (LoF) of a specific protein – 3 frameshift indels and 6 premature stop codons (Table 1 and Fig. 1 ). Eleven of the 76 protein-altering variants, including 1 LoF variant, do not fall within a previously reported locus with respect to the trait of interest. Fig. 1: Protein-altering variants with effect on lipid and liver-related blood traits. Smile plot comparing the frequency of the blood-trait increasing allele with the allele’s effect size for protein-altering variants significantly ( P < 5 × 10 −8 ) associated with a lipid (HDL-C, LDL-C, TG, TC) or liver (ALT, ALP, AST, GGT) trait. The most significant trait is shown for variants with significant association for multiple traits. Color indicates the trait category for which the variant is significant, with loss-of-function variants shown as x. Power curve (dashed line) denotes estimated 90% power in the meta-analysis with a sample size of N = 210,000 at alpha = 5 × 10 −8 . Full size image Loss-of-function variants with impact on liver-related blood traits After combining results across all samples and discovery strategies, we were particularly interested in 9 variants annotated to result in LoF of a gene. This included the not previously reported association between ZNF529 :p.K405X and decreased LDL-C, which we identified in Norwegian samples via sequencing and custom content genotyping (Table 1 ). We observed 4 additional LoF variants also resulting in substantially decreased LDL-C (3 nonsense variants in APOB , and a common frameshift indel in SLC22A1 ; Table 1 ). The 4 remaining LoF variants are associated with other blood lipid traits ( LPL :p.S474X with TG, HBB :p.Q40X with TC, and LIPC :p.G247Afs*11 with HDL-C) or ALP ( GPLD1 :p.V815Sfs*46). The previously reported LPL :p.S474X (also known as p.S447X) [17] , [18] is, in contrast to other stop-gain variants in the lipoprotein lipase ( LPL ) gene, known to result in gain-of-function of LPL [19] . This explains the association with decreased TG and points to LPL activation as a potential mechanism of CVD risk reduction. Of the 9 predicted LoF variants, the 4 within LPL , LIPC , and ZNF529 were not even nominally significantly associated ( P > 0.05) with ALT, AST, ALP or GGT (Fig. 2 ). Although we observed two very rare non-coding variants in proximity to ZNF529 that are associated with increased ALT (Supplementary Data 2 - 3 and Supplementary Fig. 5 ), these variants are completely independent ( r 2 < 0.01) of ZNF529 :p.K405X. Altogether, association results for liver enzymes and blood lipids indicate that hemizygous loss-of-function alleles in LIPC and ZNF529 and gain-of-function alleles in LPL do not cause liver damage, prioritizing these genes as potential drug targets to reduce blood lipids and CVD without liver-damaging side effects. Fig. 2: Prioritizing drug targets based on lipid effect and liver enzyme associations. For any variant significantly ( P < 5 × 10 −8 ) associated with a lipid trait (HDL-C, LDL-C, TG, TC), the maximum effect size in terms of the allele associated with good lipid health (e.g., lowered LDL-C, increased HDL-C, lowered TG, and lowered TC) is compared to the minimum p value for association with liver trait (ALT, ALP, AST, GGT). Vertical whiskers represent 95% confidence intervals of the effect size. Nominal P value of 0.05 (vertical dashed line) is indicated to highlight variants in the bottom right quadrant which lack significance for association with liver traits. These variants are better drug target candidates given estimated favorable lipid-effects on health and absence of association with potentially unfavorable liver traits. Full size image Functional characterization of ZNF529:p.K405X We expect that protein-altering variants that are the most strongly associated variants in a region represent functional variants that pinpoint biologically relevant genes and potential drug targets. We also sought not previously described genes that decreased cardiovascular risk factors (such as LDL-C) without increasing risk of liver disease or impact liver enzymes. Thus, we focused on the not previously reported association between ZNF529 :p.K405X and LDL-C (beta −0.6, P = 1.3 × 10 −8 ) since this variant is neither associated with liver enzymes ( P = 0.4−0.9 for all 4 liver enzyme traits, N range 21,530–48,569) nor non-fasting blood glucose ( P = 0.93, N = 54,093 individuals) in HUNT. Zinc finger 529 (ZNF529) does not have a homolog in rodents. To experimentally assess the consequence of ZNF529 LoF on cholesterol metabolism, we transiently knocked-down ZNF529 in human hepatoma HepG2 cells using siRNA (90.1% reduction, P = 2.7 × 10 −8 , Fig. 3a , Supplementary Data 6 ) and conducted an unbiased analysis of gene expression using RNA sequencing. Principal component analysis revealed a distinct gene expression pattern in HepG2 cells following ZNF529 knockdown with a total of 476 differentially expressed genes identified (Supplementary Fig. 6 ), including a significant upregulation of the LDL receptor (LDLR, FDR = 7.8 × 10 −7 ) (Supplementary Data 7 ). Pathway analysis revealed enrichment of general metabolism pathways, drug metabolism pathways, and lipid-related pathways (statin pathway, plasma lipoprotein remodeling and plasma lipoprotein assembly, remodeling, and clearance, P = 6.5 × 10 −4 , P = 2.2 × 10 −2 , and P = 3.9 × 10 −2 , respectively) (Supplementary Data 8 ). We confirmed the upregulation of LDLR mRNA by qPCR (90.6% increase, P = 2.9 × 10 −8 , Fig. 3b , Supplementary Data 9 ) and protein by western blot (83.0% increase, P = 0.001, Fig. 3c, d , Supplementary Data 10 ). Fig. 3: ZNF529 silencing induces LDLR expression and LDL uptake. a Efficient silencing of ZNF529 in HepG2 cells via siRNA as shown by qPCR using GAPDH as reference ( N = 21 biologically independent samples). b ZNF529 silencing in HepG2 cells induces LDLR mRNA as shown by qPCR using GAPDH as reference ( N = 21 biologically independent samples), and ( c and d ) LDLR protein as shown by western blot using β-actin as loading control ( N = 4 biologically independent samples). e ZNF529 silencing in HepG2 cells increases LDL uptake as evidenced by enhanced fluorescence of DiI-LDL (10 µg/ml, N = 9 biologically independent samples) which is inhibited in cells preloaded with 25-fold excess amounts of unlabeled-LDL (250 µg/ml, N = 3 biologically independent samples, scale bars = 200 µm), and ( f ) leads to increased intracellular cholesterol ( N = 12 biologically independent samples). Values are presented as mean ± SD (vertical whiskers) showing all points and P values (two-tailed). Mann–Whitney U test was used for a , b and f . Student t test was used for d . Source data are provided as a Source Data file. Full size image We used 1,1’-dioctadecyl- 3,3,3’,3’-tetramethylindocarbocyanine perchlorate (DiI)-labeled LDL to assess the effects of ZNF529 LoF on LDL uptake in HepG2 cells. First, we confirmed that DiI-LDL is taken-up by the cells in a dose-dependent manner, resulting in saturated uptake at 25 μg/ml (Supplementary Fig. 7 ). Next, we assessed the specificity of the binding in competition experiments between DiI-labeled and unlabeled LDL. Pretreatment of cells with 25-fold excess amounts of unlabeled LDL inhibited the uptake of DiI-LDL (Fig. 3e , Supplementary Fig. 8 ). After confirming dose-dependent saturation and specificity, we evaluated the effects of ZNF529 silencing on LDL uptake. We found that ZNF529 silencing resulted in a marked increase in DiI-LDL uptake by HepG2 cells which was suppressed in the presence of excess amounts of unlabeled LDL (Fig. 3e ). Additionally, we noted a 2.2-fold increase in intracellular cholesterol following ZNF529 knockdown ( P = 0.008, Fig. 3f , Supplementary Data 11 ). Altogether, these findings suggest that ZNF529 is a regulator of plasma LDL-C via upregulation of hepatic LDLR and enhanced LDL uptake. Clinical implications of ZNF529:p.K405X Individuals heterozygous for ZNF529 :p.K405X ( N = 109, minor allele frequency of 0.1%) had a mean LDL-C level of 2.58 mmol/L (99.8 mg/dL) vs. 3.44 mmol/L (133.0 mg/dL) in non-carriers. This reduction in LDL-C of 25% in heterozygous carriers is in the range of what is seen for treatment with 40 mg of statin [20] , and usually corresponds to a relative risk reduction of major cardiovascular events by 20–25% [2] . We only observed one homozygous female carrier. Despite being obese and hypertensive, she was alive at age >90 years and had no diagnosis of cardiovascular disease, liver disease, or diabetes, and had an LDL-C level slightly below average for her age group (3.45 mmol/L [133.4 mg/dL] vs. mean 3.8 mmol/L [147.0 mg/dL] for women >90 years old). This one individual with a natural absence of both copies of ZNF529 suggests that homozygous knockout of this gene is compatible with survival. We sought to replicate ZNF529:p.K405X outside the HUNT Study, but found that the allele count was too low for meaningful association analyses (e.g., 1 copy in 26,638 alleles in the Michigan Genomics Initiative [MGI] and 1 copy in 125,568 alleles in TOPMed). The existence of ZNF529:p.K405X in HUNT was confirmed by Sanger sequencing of the homozygous sample and 9 heterozygous samples (100% match between genotyping and Sanger sequencing) (Supplementary Fig. 9 ). Highlight of protein-altering variants with high effect size We highlight 17 protein-altering variants with an impact >1 standard deviation on the trait (Fig. 1 and Supplementary Data 12 ). For lipids, protein-altering variants in APOB, LDLR , and PCSK9 that impact LDL-C, and in CETP that impact HDL-C, are well known [17] . However, for liver enzyme traits, TNK1 :p.G574V is a new finding to complement genes previously known to impact or encode liver enzymes including ALPL (with ALP) [21] , GPLD1 (with ALP), and GPT (with ALT) [22] . This rare TNK1 variant, present in 46 individuals (1 in 814 individuals), was first identified in Norwegian sequenced samples, then genotyped using the custom array, and observed to have a large impact on ALP (beta = 1.2, P = 1.7 × 10 −14 ). Gene-based burden tests Gene-based burden results are, in contrast to single variant tests, independent of nearby signals and may point to the functional gene in a region. To identify genes functionally involved in the 9 liver-related blood traits, we performed gene-based burden tests using SKAT-O as implemented in SAIGE-GENE [23] . We included all protein-altering variants with frequency below 0.5% in the HUNT dataset. Although we found 33 unique genes to be significantly associated ( P < 2 × 10 −7 ) with at least one of 9 liver traits (Supplementary Data 13 ), in only two cases was the gene-based evidence for association substantially stronger than the strongest single variant. This comprised 10 variants in the gene GPT associated with ALT ( P = 2.35 × 10 −60 vs. P = 6.43 × 10 −25 for rs147998249) and 6 variants in the gene ALPL associated with ALP ( P = 2.9 × 10 −239 vs. P = 3.99 × 10 −67 for rs138587317). These data suggest there are multiple, functional coding rare variants in each of these two genes. 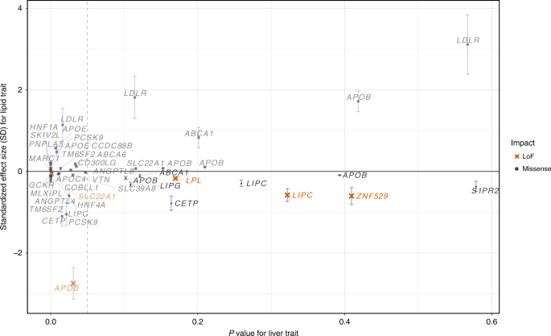Fig. 2: Prioritizing drug targets based on lipid effect and liver enzyme associations. For any variant significantly (P< 5 × 10−8) associated with a lipid trait (HDL-C, LDL-C, TG, TC), the maximum effect size in terms of the allele associated with good lipid health (e.g., lowered LDL-C, increased HDL-C, lowered TG, and lowered TC) is compared to the minimumpvalue for association with liver trait (ALT, ALP, AST, GGT). Vertical whiskers represent 95% confidence intervals of the effect size. NominalPvalue of 0.05 (vertical dashed line) is indicated to highlight variants in the bottom right quadrant which lack significance for association with liver traits. These variants are better drug target candidates given estimated favorable lipid-effects on health and absence of association with potentially unfavorable liver traits. The gene-based burden test also identified well-known genes such as CETP and ABCA1 associated with HDL-C; PCSK9, LDLR and APOB associated with LDL-C; the CRP gene associated with CRP; and GPLD1 associated with ALP (Supplementary Data 13 ). Additionally, burden tests for the 3 LoF APOB variants indicated no association with liver enzymes for heterozygous LoF carriers (Supplementary Data 14 ), highlighting APOB as another potentially valuable pharmaceutical target for blood lipid lowering. Cross-trait analyses for evaluating potential consequences of gene targeting To expand our understanding of the 76 presumed causal protein-altering variants, to investigate their impact on disease, and to evaluate potential consequences of targeting the implicated gene or its gene product, we imputed the TOPMed reference panel into the UK Biobank and performed a phenome-wide association study (PheWAS) across 1342 ICD code-defined disease groups [24] , [25] , in 408,961 people of white British ancestry. Sixty-four of the 76 protein-altering variants could be imputed sufficiently well ( R 2 > 0.3). Of 64 variants assessed, we found that 24 variants are associated with one or more diseases at a phenome-wide significance level ( P < 3.5 × 10 −5 ) (Fig. 4 , Supplementary Fig. 10 , and Supplementary Data 15 ). Fig. 4: Phenome-wide association study in UK Biobank ( N = 408,961 participants) based on presumed causal protein-altering variants with impact on liver-related blood traits in The HUNT Study ( N = 69,479). The figure displays phenome-wide statistically significant ( P < 3.5 × 10 −5 ) associations between selected protein-altering variants ( n = 21) with impact on one or more of the 9 liver-related blood traits and selected cardiovascular, liver, and metabolic phenotypes derived from ICD codes in UK Biobank. Arrows denote the direction of effect for the minor allele. Larger arrows signify more significant associations. Statistically insignificant associations are not displayed. Please see Supplementary Fig. 10 and Supplementary Data 15 for the full phenome-scan across all traits and variants available for testing in UKB ( n = 24). The ZNF529 LoF variant could not be imputed into the UK Biobank. Full size image To identify potentially useful pharmaceutical strategies that may reduce blood lipid levels and risk of coronary artery disease (CAD) and type 2 diabetes (T2D) without increasing the risk of fatty liver disease, we attempted to identify variants that decreased LDL-C or TG and decreased the risk of cardio-metabolic disease, but were not associated with changes in liver enzyme levels ( P > 0.05, Figs. 2 , 4 , Supplementary Fig. 10 and Supplementary Data 12 – 15 ), suggesting that liver function was not altered. The 2 variants with this pattern of association include (i) COBLL1 :p.N497D which is associated with decreased TG levels and decreased risk of T2D in both HUNT and UK Biobank and of liver disease in HUNT and (ii) LPL :p.S474X which is associated with decreased risk of CAD, T2D, and hypertension. HDL-C-associated ANGPTL4 p.E40K appears to decrease risk of T2D, CAD, and hypertension but is also associated with an increased risk of ankylosing spondylitis (Supplementary Fig. 10 and Supplementary Data 15 ), hence a potential complication of targeting this gene. From the PheWAS, we observed other interesting associations. For example, we found that the variant SERPINA1 :p.E366K, which is known to cause alpha-1-antitrypsin deficiency, often complicated by severe liver and pulmonary disease [26] , is also associated with a decreased risk of myocardial infarction. This finding supports clinical evidence that individuals with alpha-1-antitrypsin deficiency may be protected against coronary artery disease [27] . The association, however, also suggests caution in ongoing efforts to treat acute myocardial infarction with exogenous administration of alpha-1-antitrypsin [28] , [29] , because the genetic association suggest the opposite effect – an increased risk of myocardial infarction. Another interesting finding is the low-frequency S1PR2 variant p.Y257C (chr19:10224136T>C, MAF = 0.003) which we found to be associated with decreased LDL-C (effect of -0.37 SD, P = 6 × 10 −9 ) and a decreased risk of coronary artery disease, including myocardial infarction (odds ratio 0.45, P = 0.0005), without being associated with liver enzyme traits (Supplementary Data 12 ). Further studies are obviously warranted to uncover the biological mechanisms underlying the associations described here, however, each of them could help inform clinical implications of targeting the underlying gene or gene product. By using complementary approaches for genomic association discovery: sequencing, imputation, array-based genotyping, stepwise conditional analyses and trans-ancestry meta-analyses, we identified >650 independent genomic variants associated with quantitative liver-related disease precursors. This included 76 protein-altering variants that we assume to be causally related to one or more of the traits. By broadly considering associations between these protein-altering variants, quantitative traits, and disease endpoints, we prioritize several genes as potential pharmaceutical targets for preventing or treating CVD. The newly uncovered association and in vitro studies indicate that ZNF529 LoF is associated with lower plasma LDL-C, which could be explained by induction of LDLR in hepatic cells and increased LDL uptake. While these findings indicate a therapeutic potential for lowering plasma LDL-C by ZNF529 inhibition, further studies are warranted to elucidate the mechanisms by which ZNF529 regulates LDLR and LDL uptake in the liver. Considering that ZNF529 does not have a homolog in rodents, the use of animal models for such studies is limited. Another interesting finding to highlight is the presumed causal low-frequency protein-altering variant S1PR2 :p.Y257C that we found to be associated with decreased LDL-C and a >50% reduction in the risk of myocardial infarction, without being associated with altered liver function or non-fasting blood glucose. 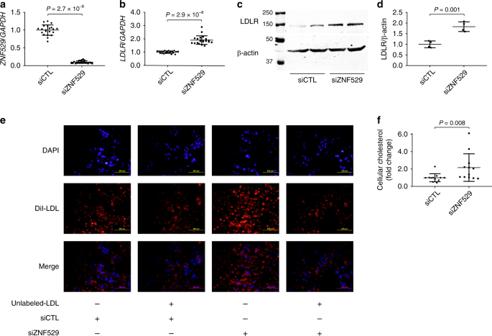Fig. 3: ZNF529 silencing induces LDLR expression and LDL uptake. aEfficient silencing of ZNF529 in HepG2 cells via siRNA as shown by qPCR using GAPDH as reference (N= 21 biologically independent samples).bZNF529 silencing in HepG2 cells induces LDLR mRNA as shown by qPCR using GAPDH as reference (N= 21 biologically independent samples), and (candd) LDLR protein as shown by western blot using β-actin as loading control (N= 4 biologically independent samples).eZNF529 silencing in HepG2 cells increases LDL uptake as evidenced by enhanced fluorescence of DiI-LDL (10 µg/ml,N= 9 biologically independent samples) which is inhibited in cells preloaded with 25-fold excess amounts of unlabeled-LDL (250 µg/ml,N= 3 biologically independent samples, scale bars = 200 µm), and (f) leads to increased intracellular cholesterol (N= 12 biologically independent samples). Values are presented as mean ± SD (vertical whiskers) showing all points andPvalues (two-tailed). Mann–WhitneyUtest was used fora,bandf. Studentttest was used ford. Source data are provided as a Source Data file. 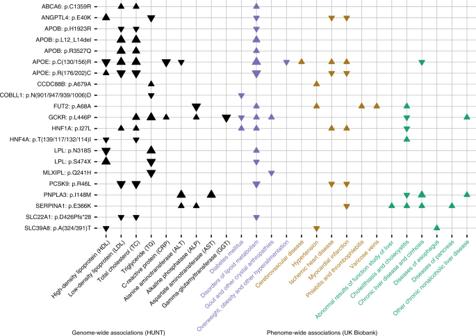Fig. 4: Phenome-wide association study in UK Biobank (N= 408,961 participants) based on presumed causal protein-altering variants with impact on liver-related blood traits in The HUNT Study (N= 69,479). The figure displays phenome-wide statistically significant (P< 3.5 × 10−5) associations between selected protein-altering variants (n= 21) with impact on one or more of the 9 liver-related blood traits and selected cardiovascular, liver, and metabolic phenotypes derived from ICD codes in UK Biobank. Arrows denote the direction of effect for the minor allele. Larger arrows signify more significant associations. Statistically insignificant associations are not displayed. Please see Supplementary Fig.10and Supplementary Data15for the full phenome-scan across all traits and variants available for testing in UKB (n= 24). The ZNF529 LoF variant could not be imputed into the UK Biobank. The variant was identified via low-pass sequencing and custom content genotyping in HUNT. S1PR2 encodes sphingosine-1-phosphate receptor 2, which seems to play a critical role in the endothelial inflammatory response [30] . Several animal models have already indicated that inhibition of S1PR2 could be a valuable pharmaceutical target for vascular recovery in coronary artery disease and stroke [30] , [31] , [32] . The associations that we report here represent the first direct human data supporting that S1PR2 might play an important role in ischemic heart disease. Taken together, we demonstrate that identifying rare protein-altering variants and careful consideration of multiple phenotypes in well-powered studies may point to promising pharmaceutical drug targets. We used a variety of approaches to identify rare protein-altering variants, and we found that if exome sequencing is prohibitively expensive, sequencing a subset of samples followed up with a custom genotyping array can be a viable strategy to identify impactful rare variants. The HUNT Study The Trøndelag Health Study (HUNT) is a population-based health survey conducted in the county of Trøndelag, Norway, since 1984 [9] . Participation in the HUNT Study is based on informed consent and the study has been approved by the Data Inspectorate and the Regional Ethics Committee for Medical Research in Norway (REK: 2014/144). We included a total of 69,479 individuals with values for at least one of the traits examined (ALT, ALP, AST, CRP, GGT, HDL-C, LDL-C, TC and TG). Genotyping was performed using the Illumina Human CoreExome v1.1 array with 70,000 additional custom content beads [33] , [34] . Variants were selected for genotyping if they were: protein-altering ( n = 13,618); modestly associated with lipids in HUNT but not tested in large consortia ( n = 960); identified as causing familial hypercholesterolemia in Norwegian patients ( n = 110); or predicted to result in a loss-of-function of one of the 56 ACMG genes ( n = 27,144, Supplementary Data 16 ). Additionally, we selected missense variants with 2 or more copies ( n = 8720) and nonsense variants with 1 or more copy ( n = 756) identified from low-pass whole-genome sequencing of 2202 HUNT samples. Please see Supplementary Data 17 for a summary of selected custom content variants. Imputation was performed from 60,039 TOPMed reference genomes using Minimac3 and variants with imputation quality >0.3 were retained. To account for relatedness within the sample, we performed association testing using the linear mixed model with genetic relationship matrix as implemented in SAIGE [ https://github.com/weizhouUMICH/SAIGE ] [12] . Birth year, sex and PC1-4 were included as covariates. Conditional analysis was performed with the same analysis tools and command line options as the association analysis by adding the lead-SNP(s) in a step-wise manner as covariate(s) into the SAIGE step1 parameter estimation until the variant with smallest P value in the locus was >5 × 10 −8 . Biobank Japan Biobank Japan (BBJ) is a multi-institutional hospital-based registry of ~200,000 individuals from 66 Japanese hospitals collected from 2003 to 2007. ﻿Written informed consent was obtained from all participants, as approved by the ethics committees of RIKEN Center for Integrative Medical Sciences and the Institute of Medical Sciences, the University of Tokyo. Genotype, imputation, and QC were performed as described previously [14] . Briefly, samples were genotyped with Illumina HumanOmniExpressExome or a combination of the Illumina HumnOmniExpress and HumanExome BeadChips and imputed using 1000 Genomes Project Phase 1 version 3 East Asian reference haplotypes. Publicly available summary statistics from linear regression assuming an additive model for quantitative measures of ALP, ALT, AST, CRP, GGT, HDL-C, LDL-C, TC, and TG were used. Quantitative traits were adjusted for age, sex, top 10 PCs of genetic ancestry, and disease status for 47 target diseases. Sample sizes for traits ranged from 70,567 to 134,182 [14] . SardiNIA 6602 individuals from four villages in the Lanusei valley on Sardinia (>60% of the adult population) were genotyped on four different Illumina Infinium arrays: OmniExpress, Cardio-Metabochip [35] , Immunochip [36] , and Exome Chip. Low-depth (~4x coverage) whole-genome sequencing on 3839 individuals was performed, of which 2340 were also genotyped. Imputation of 1.1 million indels and 24.1 million biallelic single nucleotide variants was performed using Minimac3 [37] and markers with imputation quality >0.3 (or >0.6 if MAF<1%) were retained. Samples, genotyping, sequencing and variant calling have been previously described [38] . Liver traits (ALT, AST, CRP, GGT, HDL-C, TC, and TG) from the first visit were used and LDL-C was computed using the Friedewald Equation [13] . Association analyses were performed for liver traits assessed in 5570–5942 individuals (median N = 5917) using age, age 2 and sex-adjusted inverse-normalized residuals of the outcomes as input to the Efficient Mixed Model Association eXpedited (EMMAX) [39] single variant test (i.e., a linear model with a kinship matrix) as implemented in EPACTS [ https://github.com/statgen/EPACTS ]. Genomic control correction was not applied as the lambda values were not inflated (range 0.97–1.02, Supplementary Data 18 ). The study, including the protocols for subject recruitment and assessment, the informed consent for participants (or consent from their legally authorized representative for those 14–17y); and the overall analysis plan was reviewed and approved by institutional review boards for the Istituto di Ricerca Genetica e Biomedica (IRGB; Cagliari, Italy), for the MedStar Research Institute (responsible for intramural research at the National Institutes of Aging, Baltimore, Maryland, United States), and for the University of Michigan (Ann Arbor, Michigan, United States). Meta-analyses As the summary statistics from SardiNIA and Biobank Japan were in Human Genome Build hg19, the positions were mapped to Human Genome Build hg38 using liftOver [ https://genome.ucsc.edu/cgi-bin/hgLiftOver ]. The genomic control corrected summary statistics from the contributing cohorts were combined with METAL [40] using inverse variance weighted meta-analysis. Meta-analysis included SardiNIA, Biobank Japan, and HUNT for all traits, with the exception of ALP which was only available from HUNT and Biobank Japan. Definition of independent loci Independent loci were defined as genetic markers >1 Mb apart in physical distance with at least one genetic variant associated with the trait of interest at a genome-wide significance threshold of P < 5 × 10 −8 . Loci borders were defined as the highest and lowest genomic positions within the locus reaching genome-wide significance plus an additional 1 Mb on either side. Novelty of identified genomic loci A locus was classified as known if a variant previously published to be associated with the trait of interest fell with 1Mb of the locus lead variant that we identified. Otherwise, a locus was classified as novel. Previously published variants were extracted from papers and the GWAS catalog [https://www.ebi.ac.uk/gwas/] at the time of analyses. PheWAS in UK Biobank Association results for 1342 trait groups (PheCodes) [24] in UK Biobank were generated using SAIGE [12] . Phenotypes were grouped by combining ICD-9 and ICD-10 codes of closely related traits following previously published methods [25] . Analyses were performed on the white British subset of UK Biobank after imputation with the TOPMed reference panel. Sex, birth year, and 4 principal components were included as covariates. Significance was determined based on Bonferroni correction for the number of traits tested ( P < 3.5 × 10 −5 ). Participation in the UK Biobank is based on informed consent [41] . Gene-based SKAT-O tests The exome-wide gene-based SKAT-O tests were performed using SAIGE-GENE v36 [23] for all 9 liver traits based on the TOPMed-imputed HUNT data. Missense and stop-gain variants annotated by ANNOVAR [42] with MAF ≤ 0.005 were included. Conditional analyses were performed to condition on the most significant single variant association signal within 500 kB of the gene. We selected a significance threshold of 2.5 × 10 −6 accounting for 20,000 genes. Replication attempt of ZNF529:p.K405X in MGI The Michigan Genomics Initiative (MGI) is a repository of electronic medical record and genetic data at Michigan Medicine (N~58,000 participants). MGI participants were enrolled during pre-surgical encounters at Michigan Medicine and provided consent to study genetic and electronic health record data for research. The MGI study was approved by the Institutional Review Board of the University of Michigan Medical School. DNA was extracted from blood samples and participants were genotyped using Illumina Infinium CoreExome-24 bead arrays, which includes the same custom content as the HUNT Study. Genotype data were imputed to the Haplotype Reference Consortium using the Michigan Imputation Server, providing 17 million imputed variants after standard quality control and filtering. Only European individuals were used for analysis. We attempted to replicate the association with ZNF529:p.K405X in 13,319 MGI participants with LDL-C measurements, however, only 1 participant was heterozygous for ZNF529:p.K405X so the power to detect association was near zero. In contrast, we identified 110 heterozygous individuals in the HUNT discovery study. HepG2 cells The HepG2 human hepatoma cell line was obtained from the American Type Culture Collection (ATCC) and cultured at 37 °C and 5% CO 2 in Dulbecco’s Modified Eagle Medium (DMEM, Gibco) supplemented with 10% fetal bovine serum (FBS, Sigma-Aldrich) and 1% Penicillin-Streptomycin (Pen-Strep, Gibco). ZNF529 gene silencing using small interfering RNA (siRNA) siRNA targeting zinc finger protein 529 (siZNF529: GGCUUUUGGAGUAUGUAGAtt) and non-targeting siRNA control (siCTL) were obtained from Ambion (siRNA IDs s33654 and AM4611, respectively). HepG2 cells were transfected with 20 nM of siZNF529 or siCTL using Lipofectamine RNAiMAX (Invitrogen) in Opti-MEM reduced-serum medium (Gibco) in accordance with the manufacturer’s protocol [43] . Cellular lipid or protein extraction, RNA isolation or LDL uptake assays were conducted 48 h post transfection. RNA sequencing Total RNA was purified from HepG2 cells using the QIAGEN’s RNeasy kit (QIAGEN). Library preparation and sequencing were performed by the University of Michigan DNA Sequencing Core. RNA was assessed for quality using the TapeStation (Agilent, Santa Clara, CA). All samples had RNA integrity numbers (RINs) >8.5. Samples were prepared using the NEBNext Ultra II Directional RNA Library Prep Kit for Illumina (NEB, E7760L) with Poly(A) mRNA Magnetic Isolation Module (NEB, E7490L) and NEBNext Multiplex Oligos for Illumina Unique dual (NEB, E6440L), where 10 ng–1 µg of total RNA were subjected to mRNA polyA purification. The mRNA was then fragmented and copied into first strand cDNA using reverse transcriptase and dUTP mix. Samples underwent end repair and dA-Tailing step followed by ligation of NEBNext adapters. The products were purified and enriched by PCR to create the final cDNA library. Final libraries were checked for quality and quantity by TapeStation (Agilent) and qPCR using Kapa’s library quantification kit for Illumina Sequencing platforms (Kapa Biosystems, KK4835). Libraries were paired-end sequenced on a NovaSeq 6000 Sequencing System (Illumina). Paired-end reads (101 bp) from RNA sequencing of 4 siCTL and 4 siZNF529 samples were aligned to hg38 reference genome using Tophat2 (v2.0.13 11/5/19 7:29:00 PM) [44] with default parameters. In each sample, 94.3–95.4% reads could be aligned. All valid alignments were used for downstream analysis. GENCODE release 29 was used to obtain gene boundaries of 19,940 protein coding genes. We used Samtools (v1.9) [45] and bedtools (v2.22.0) [46] coverage function to count number of reads aligned in each genic bin. Genes with >3 counts per million (CPM) in 8 samples were used for further analysis. EdgeR [47] library in R was used to identify differentially expressed genes (Supplementary Data 7 ). We used glmFit followed by glmTreat to identify significant change in expression with FDR < 0.05. We used ConsensusPathDB [48] to identify enriched pathways from list of differentially expressed genes (Supplementary Data 8 ). RNA isolation, RT-PCR and qPCR Total RNA was purified from HepG2 cells using the QIAGEN’s RNeasy kit (QIAGEN). cDNA was synthesized using SuperScript III (Invitrogen), and qPCR was performed using SYBR green reagents (Bio-Rad). Gene expression is presented as fold-change compared with RNA isolated from control cells by the comparative CT (2 −ΔΔCT ) method using GAPDH as the reference gene [49] , [50] . Primer pairs used for qPCR were obtained from Integrated DNA Technologies and are available in Supplementary Data 19 . Protein extraction and western blot Cells were lysed in radioimmunoprecipitation assay lysis buffer (RIPA buffer, Thermo Scientific) supplemented with a protease inhibitor cocktail (Roche Applied Science). Proteins were resolved in 8% sodium dodecyl sulfate polyacrylamide gel electrophoresis (SDS-PAGE) and transferred to nitrocellulose membranes (Bio-Rad). The membranes were blocked for 1 h at room temperature in tris-buffered saline-Tween 20 (TBST) containing 5% fat-free milk and incubated with primary antibody at 4 °C overnight. The following primary antibodies were used: rabbit monoclonal anti-LDLR antibody (Abcam, ab52818, working dilution 1:1000) and mouse monoclonal anti-β-actin antibody (Cell signaling, 8H10D10, working dilution 1:2000). After TBST washing, membranes were incubated with secondary antibodies (LI-COR Biotechnology, donkey anti-rabbit IRDye 926-32213 and donkey anti-mouse IRDye 926-68072, working dilution 1:10000) for 1 h at room temperature. After TBST washing, bands were visualized and quantified using an Odyssey Infrared Imaging System (LI-COR Biosciences, version 2.1) [49] . DiI-LDL uptake assay 1,1’-dioctadecyl- 3,3,3’,3’-tetramethylindocarbocyanine perchlorate-low-density lipoprotein (DiI-LDL Alfa Aesar, J65330 or Kalen Biomedical, 770230-9) was used to evaluate the cellular uptake of LDL [51] in accordance with the manufacturer’s instructions. Briefly, 48 h following siRNA transfection, HepG2 cells were washed with PBS (x2) and changed to serum-free DMEM supplemented with 0.1% bovine serum albumin (BSA, Sigma-Aldrich). The cells were then incubated with DiI-LDL (1–25 μg/ml) for 5 h at 37 °C in the dark. In some experiments, cells were pre-treated for 30 min with 25-fold excess amounts of unlabeled LDL (Alfa Aesar, J65039) to assess the specificity of the binding. Nuclei were stained with 4′,6-diamidino-2-phenylindole (DAPI, Cayman Chemical Company, 14285). After incubation, the cells were washed with PBS (x2) and changed to serum- and probe-free DMEM. Finally, the cells were visualized using a fluorescent microscope (Olympus, IX71). For each experiment two random fields were chosen and photographed in a blinded fashion. DiI-LDL and DAPI images were merged using ImageJ software (v.1.52k, NIH). Lipid extraction and cholesterol quantification The lipids of HepG2 cells were extracted using hexane (≥99%, 32293, Sigma-Aldrich) and isopropanol (≥99.5%, A426-4, Fisher Chemicals) at a 3:2 ratio ( v:v ), and the hexane phase was left to evaporate for 48 h. The remaining cells in the plates were disrupted in 0.1 M NaOH for 24 h and an aliquot was taken for measurement of cellular protein using the Bradford protein assay (Bio-Rad). The content of cellular cholesterol was determined spectrophotometrically using a commercially available kit (Wako Chemicals, 999-02601). Cholesterol data were normalized to cellular protein levels [49] , [52] . Statistical analyses for in vitro studies Statistical analyses were performed using SPSS 24.0 software (SPSS Inc. IBM). Unless indicated otherwise, values are presented as mean ± SD showing all points. All data were tested for normality and equal variance. If the data passed those tests, Student t test was used for comparisons between the two groups. If the data did not pass those tests, nonparametric Mann–Whitney U test was used. P < 0.05 was considered statistically significant. Reporting summary Further information on research design is available in the Nature Research Reporting Summary linked to this article.